High-sensitivity linear piezoresistive transduction for nanomechanical beam resonators Highly sensitive conversion of motion into readable electrical signals is a crucial and challenging issue for nanomechanical resonators. Efficient transduction is particularly difficult to realize in devices of low dimensionality, such as beam resonators based on carbon nanotubes or silicon nanowires, where mechanical vibrations combine very high frequencies with miniscule amplitudes. Here we describe an enhanced piezoresistive transduction mechanism based on the asymmetry of the beam shape at rest. We show that this mechanism enables highly sensitive linear detection of the vibration of low-resistivity silicon beams without the need of exceptionally large piezoresistive coefficients. The general application of this effect is demonstrated by detecting multiple-order modes of silicon nanowire resonators made by either top-down or bottom-up fabrication methods. These results reveal a promising approach for practical applications of the simplest mechanical resonators, facilitating its manufacturability by very large-scale integration technologies. Doubly clamped beams based on nanostructures such as carbon nanotubes (CNTs) [1] and silicon nanowires (SiNWs) [2] , [3] are excellent building blocks for the realization of nanomechanical resonators with ultra-high-performance characteristics. Such devices have provided functional features at the verge of fundamental limits in several contexts, ranging from physical sensing [4] , [5] , [6] to signal processing [7] , [8] . CNT resonators are at the forefront of recent advances in extreme performance, but their unique features degrade drastically at room temperature [9] . Moreover, CNT device fabrication technologies are still far from the large-scale/high-yield production requirements for real-world applications. On the other hand, SiNW resonators have shown lower performance levels but better possibilities for room temperature operation. And a doubly clamped SiNW resonator is the simplest resonant nanostructure that can be monolithically fabricated. This structural simplicity enables their fast, reproducible and low-cost fabrication by very large-scale integration (VLSI) methods at the wafer scale [10] . However, one of the most limiting difficulties for the practical development of batch-fabricated SiNW resonators with performance characteristics approaching those of CNTs is to establish highly sensitive transduction schemes that efficiently convert mechanical vibrations into functional electrical signals. The small amplitude of the mechanical vibrations, in combination with their very high frequency and the natural tendency of high-aspect ratio beams to operate in a nonlinear regime, represents formidable obstacles for such purpose [11] , [12] . The application of the most sensitive transduction schemes reported so far for nanomechanical resonators, such as piezoelectric [13] , electrothermal [14] or optomechanical [15] , results either impossible or impractical for simple beams made of silicon with dimensions deep down in the nanoscale and resonant frequencies in the very high-frequency range. Electromechanical transduction is the alternative of choice whenever nanomechanical resonators can benefit from integration with on-chip electronics that incorporate additional functions. Integration allows multiplexing, signal conditioning and amplification, facilitates portability and enables multi-sensing platforms [16] . In general, different mechanisms can be used for electromechanical transduction. For CNT resonators, the most widely used method is modulation of the CNT conductivity induced by capacitive coupling with a gate located at close proximity [1] , requiring the use of semiconducting CNTs. The measurement of capacitance variation of the oscillating structure with respect to a fixed electrode has also been widely used in silicon-based mesoscopic resonators [17] , [18] . However, this approach presents enormous difficulties for very small devices. It requires the realization of very small actuation/read-out gaps, and even then, the minuscule change in motional capacitance to be measured is hindered by parasitic capacitances. Although modulation of the conductivity by capacitive transduction can also be implemented in SiNW resonators [3] , [19] , piezoresistive transduction offers a more straightforward solution a priori , as silicon is a piezoresistive material. For example, piezoresistive transduction has been implemented in U-shaped micromechanical resonators with longitudinal resonant modes over 1 GHz (ref. 20 ). For the case of doubly clamped SiNW resonators, the whole beam body can operate as a piezoresistive gauge for flexural modes, so that transduction is provided by the change of resistance of the beam induced by its periodic elongation as it vibrates ( Fig. 1 ). Nevertheless, the minute amplitude typically produced for the mechanical vibration implies that this elongation is too small to result in signals that can be measured by simple means if the piezoresistive coefficients of bulk Si are considered. However, the piezoresistive coefficients of Si have been found to increase considerably in bottom-up-synthesized SiNWs [21] . In addition, anomalously enhanced piezoresistive behaviour in highly strained, undoped SiNWs has been reported [22] . The so-called giant piezoresistance effect has indeed been explored for electrical read-out of high-frequency SiNW resonators [2] . Several studies in top-down SiNWs have not been able to find giant values of piezoresistance coefficients [23] , [24] . 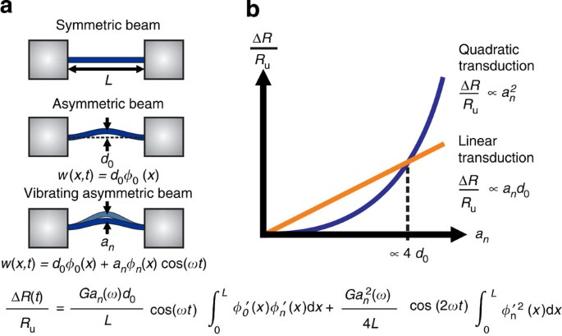Figure 1: Modelling of piezoresistive transduction in doubly clamped beam nanomechanical resonators. (a) Vibrating beam with asymmetric deflection profile at rest: the overall deflectionw(x,t) is given by the sum of a deflection profile at restφ0(x) normalized to a maximum deflectiond0and a vibration deflection profileφn(x) for thenth-order mode normalized to a maximum amplitudean. (b) Relation between the relative change of resistance (ΔR/Ru,Rubeing the undeflected beam resistance) and the amplitude of vibrationan: the two curves represent the linear and quadratic components of the piezoresistive transduction. The plot shows that for vibration amplitudes smaller than the maximum deflection at rest (an<4d0), the linear component is larger than the quadratic one. Figure 1: Modelling of piezoresistive transduction in doubly clamped beam nanomechanical resonators. ( a ) Vibrating beam with asymmetric deflection profile at rest: the overall deflection w ( x , t ) is given by the sum of a deflection profile at rest φ 0 ( x ) normalized to a maximum deflection d 0 and a vibration deflection profile φ n ( x ) for the n th-order mode normalized to a maximum amplitude a n . ( b ) Relation between the relative change of resistance (Δ R / R u , R u being the undeflected beam resistance) and the amplitude of vibration a n : the two curves represent the linear and quadratic components of the piezoresistive transduction. The plot shows that for vibration amplitudes smaller than the maximum deflection at rest ( a n <4 d 0 ), the linear component is larger than the quadratic one. Full size image In this communication we describe a physical mechanism that provides highly sensitive and linear piezoresistive transduction for Si beam resonators. This mechanism enables detection of the miniscule vibration amplitude of the resonators at high frequency even in the case that the piezoresistive coefficients are comparable to those of bulk silicon. We show that when the vibration of the beam modulates the longitudinal strain with respect to an asymmetric beam shape at rest, then the piezoresistive effect originates both linear and quadratic components in the transduced signals. The transduction mechanism implies that linear transduction is largely amplified as compared with quadratic transduction depending on the magnitude of the asymmetry. This effect can be used for Si beam resonators obtained by diverse fabrication methods, as it is proved here for both bottom-up SiNW grown by the vapour–liquid–solid (VLS) mechanism and top-down SiNW defined by conventional clean-room techniques. Modelling piezoresistive transduction The emergence of amplified linear piezoresistive transduction in doubly clamped beam resonators can be demonstrated by considering the following simple model ( Fig. 1a ). We refer to electromechanical transduction as the relationship between the measured electrical signal and the mechanical vibration amplitude of the beam. We consider a single vibration mode driven at a frequency ω . Then, the beam profile at any time is assumed to be given by two contributions: first, an asymmetric deflection profile at rest as a consequence of static forces acting at the clamps resulting from the fabrication process; second, a vibration mode shape profile that is excited by the electrostatic driving force. Therefore, the beam profile can be written as: where x is the longitudinal coordinate along the beam, ω is the driving frequency, φ 0 ( x ) is the asymmetric beam profile at rest normalized to the maximum deflection at rest d 0 and φ n ( x ) is the n th-order vibration mode profile normalized to the maximum vibration amplitude of the mode a n ( ω ). We consider here that d 0 is the component of the beam deflection at rest in the vibrational plane of the corresponding mode. The piezoresistive effect implies the following relationship between the time-varying resistance change Δ R ( t ) and the total net strain ε ( t ) along the nanowire (NW) induced by the beam vibration: where R u is the undeflected beam resistance and G is the piezoresistive gauge factor. In order to calculate the strain we consider the deflection given by equation (1). The total net strain caused by the beam deflection is then given by: where prime denotes derivative with respect to the longitudinal spatial coordinate x , and L is the undeflected beam length. By combining equations (1, 2, 3), we obtain the following expression for the time-dependent components of the resistance variation (see Supplementary Discussion ): To quantify the effect of the deflection at rest and vibration profile shapes, we would need to solve the Euler–Bernouilli equation for the beam and obtain the profile shapes for a suitable set of boundary conditions. But more importantly, and regardless of the quantitative effect of the profile shapes, equation (4) shows that the time-varying resistance change has two components ( Fig. 1b ): the first one at frequency ω is proportional to the vibration amplitude times the deflection at rest (linear transduction); the second one at frequency 2 ω is proportional to the square of the vibration amplitude (quadratic transduction), and it does not depend on the deflection at rest. In addition, equation (4) also implies that the presence of a deflection at rest larger than the oscillation amplitude produces an amplification effect on the piezoresistive transduction as compared with the case of a symmetric beam shape at rest. This amplification can be expected to provide measurable electrical signals even in the case that the gauge factor is not significantly larger than that of bulk silicon. The ratio between the linear and quadratic transduction terms in equation (4) provides a measure of the gain factor of this amplification effect: We can obtain a simplified expression for this gain factor by considering a beam vibration in the fundamental mode ( n =1) and a beam deflection profile shape at rest that can be approximated by that of the fundamental mode, so that φ 0 ( x )≈ φ 1 ( x ). Then . Fabrication and characterization of the frequency response We have applied the model described above to analyse the transduction mechanism in highly doped SiNW resonators fabricated by two different methods: bottom-up fabrication by VLS growth ( Fig. 2a ); and top-down fabrication based on photolithography and standard micromachining processes, including sequential cycles of oxidation/oxide etching to reduce the SiNW diameter ( Fig. 2b ; see Methods). For both bottom-up and top-down devices, a side-gate electrode is placed in close proximity to the NW for electrostatic actuation. The resulting gap distance is around 400 nm for bottom-up devices and 900 nm for top-down devices. In both cases, the final resistivity of the SiNWs is very low in the range of 10 −4 Ω m. Each fabrication method produces particular morphological features that affect the behaviour of the SiNWs as nanomechanical resonators. Bottom-up SiNWs grow along the <111> direction and present hexagonal section, epitaxial clamps and smooth surface. Under the present growth conditions, they show a slightly tapered geometry. In the case of top-down SiNWs, their cross-section is not regular either, wider near the clamping ends due to the preference of the oxidation process for certain directions of the crystalline structure. Also, the oxidation/etching steps produce an overhanging membrane at the ends of the anchoring structures. 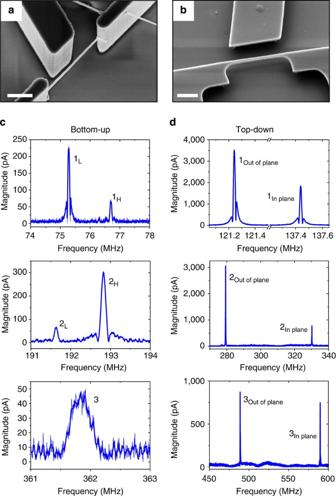Figure 2: Frequency response of SiNW nanomechanical resonators under study obtained by the FM detection method. (a) SEM image of a bottom-up growth SiNW resonator. Line scale, 500 nm. (b) SEM image of a top-down-fabricated SiNW resonator. Line scale, 1 μm. (c) Electrical measurement of the frequency response of a bottom-up resonator showing (from top-to-bottom) the first, second and third resonance modes. The NW has a length of 3 μm and a cross-sectional flat-to-flat distance of around 90 nm. The subscripts ‘L’ and ‘H’ refer to the low-frequency and high-frequency peaks of each resonant mode, corresponding to different directions of vibration. Measurement conditions for the first mode of resonance:VNW=200 mV,Vg,DC=5 V. Measurement conditions for the second mode of resonance:VNW=350 mV,Vg,DC=18 V. Measurement conditions for the third mode of resonance:VNW=1,125 mV,Vg,DC=25 V. (d) Electrical measurement of the frequency response of a top-down SiNW resonator showing (from top-to-bottom) the first, second and third resonance modes. The NW has cross-sectional dimensions of 137 nm (thickness) × 140 nm (width), and a length of 3 μm. Measurement conditions for the first mode of resonance:VNW=140 mV,Vg,DC=10 V. Measurement conditions for the second mode of resonance:VNW=250 mV,Vg,DC=15 V. Measurement conditions for the third mode of resonance:VNW=250 mV,Vg,DC=15 V. Figure 2: Frequency response of SiNW nanomechanical resonators under study obtained by the FM detection method. ( a ) SEM image of a bottom-up growth SiNW resonator. Line scale, 500 nm. ( b ) SEM image of a top-down-fabricated SiNW resonator. Line scale, 1 μm. ( c ) Electrical measurement of the frequency response of a bottom-up resonator showing (from top-to-bottom) the first, second and third resonance modes. The NW has a length of 3 μm and a cross-sectional flat-to-flat distance of around 90 nm. The subscripts ‘L’ and ‘H’ refer to the low-frequency and high-frequency peaks of each resonant mode, corresponding to different directions of vibration. Measurement conditions for the first mode of resonance: V NW =200 mV, V g,DC =5 V. Measurement conditions for the second mode of resonance: V NW =350 mV, V g,DC =18 V. Measurement conditions for the third mode of resonance: V NW =1,125 mV, V g,DC =25 V. ( d ) Electrical measurement of the frequency response of a top-down SiNW resonator showing (from top-to-bottom) the first, second and third resonance modes. The NW has cross-sectional dimensions of 137 nm (thickness) × 140 nm (width), and a length of 3 μm. Measurement conditions for the first mode of resonance: V NW =140 mV, V g,DC =10 V. Measurement conditions for the second mode of resonance: V NW =250 mV, V g,DC =15 V. Measurement conditions for the third mode of resonance: V NW =250 mV, V g,DC =15 V. Full size image For both bottom-up and top-down devices, an asymmetric beam profile at rest is observed by scanning electron microscopy (SEM) and atomic force microscopy. The magnitude of the maximum deflection d 0 varies from device to device, and the images provided in Supplementary Figs 1–3 show that it lays in the range of 5–50 nm for both types of devices. However, the maximum deflection d 0 is typically larger for top-down SiNWs, where it systematically reaches a few tens of nanometres. In this case, it is attributed to tensile stress produced by the under-etched parts of the anchoring structures that bend up during the fabrication process (see Supplementary Fig. 2 ). In the case of bottom-up NWs, the deformation has a larger device-to-device variation, and it is attributed to VLS growth effects such as secondary NW growth at the impinging end clamp [25] . The bottom-up devices used for this study had a maximum deflection d 0 always below 10 nm, although SiNWs with a much larger deflection were sometimes obtained. The electromechanical response of the fabricated devices has been characterized by three different frequency down-mixing detection methods: frequency modulation (FM) demodulation [8] , two-source/1 ω (ref. 1 ) and two-source/2 ω (ref. 2 ). Details about the experimental implementation of each detection scheme can be found in Methods. FM demodulation provides the higher signal-to-noise ratio and signal-to-background ratio measurements, and thus it is used here as the method of reference for characterizing the frequency response of the devices. Although FM demodulation has been demonstrated to provide a linear transduction component, higher-order terms may also contribute to the measured signal [8] . However, the two-source/1 ω and two-source/2 ω schemes selectively target the linear and the quadratic components of the resistance variation, respectively, so that they are used here to probe the relative magnitude of these components. Regardless of the detection method, the electromechanical characterization of the resonators shows unambiguously the position of the resonance peaks and the presence of split modes. Figure 2 shows representative examples of the frequency response of bottom-up and top-down SiNW resonators. Remarkably, the resonance peaks of Fig. 2c,d produce larger (cleaner) signals than those reported previously for SiNW resonators [2] , [3] , [19] . Besides the fundamental modes, we find it possible to detect higher-order modes, even at frequencies higher than 500 MHz, for which the vibration amplitude is expected to be very small. Figure 2c shows the frequency response of a bottom-up SiNW with a length of 3 μm and an average diameter of around 90 nm. The first three mechanical modes of resonance are detected. Each mode is split in two orthogonal modes corresponding to two preferential resonant directions, which arise from the irregular geometry of the hexagonal cross-section and other structural defects [26] . A quality factor of 3,600 is estimated for the first mode of resonance. Figure 2d shows the frequency response of a top-down SiNW resonator. We also observe the first three resonant modes, and each one is split in two orthogonal modes similarly to the bottom-up resonators. In this case, the two orthogonal modes are more separated in frequency because the cross-sectional area of the SiNW is rectangular and the radial asymmetry is larger than that of the bottom-up SiNWs. The quality factor of the first mode is around 4,900 for each of the split modes, remarkably larger than the one obtained for the bottom-up SiNWs. This indicates that the effect of the overhanging membrane in the clamping is not detrimental to obtain a good mechanical response. To our knowledge, these are the first electrical measurements obtained for the higher modes of a SiNW mechanical resonator fabricated by top-down methods at this dimensions. We performed finite element simulations using Ansys [27] to confirm that the measured resonance peaks actually correspond to the first three mechanical modes (see Supplementary Fig. 4 ). First, finite element simulations were performed for a bottom-up SiNWs mechanical resonator made of a crystalline SiNW (cross-sectional flat-to-flat distance of 90 nm, length of 3 μm) following the <111> direction and with perfect clamping to rigid side walls. Table 1 shows that the values of the experimental resonance frequencies are higher than the values obtained from the simulation when absence of stress is considered. This is an indication of the presence of stress/strain in the bottom-up SiNW resonators at rest. Table 1 Comparison between the experimental and simulated resonance frequencies for the bottom-up and top-down SiNW nanomechanical resonators of Fig. 2. Full size table The simulations are replicated in the case of SiNW mechanical resonators fabricated by the top-down method. In this case the geometry is more complex, as the resonators present a widening near the clamping and overhangs that are difficult to characterize. A model based on SEM images is built in which both of these effects are taken into account. The simulations and subsequent fitting of the longitudinal stress are performed similarly to the case of the bottom-up SiNWs. We find that the experimental frequencies are higher than the simulated ones in the absence of stress ( Table 1 ). By introducing a stress in the simulations, we find that the experimental measurements are coherent with a longitudinal tensile stress of around 500 MPa. We have used SEM imaging to estimate the actual vibration amplitude of the resonators while vibrating at resonance (see Supplementary Fig. 5 ). We find that the vibration amplitude is below the resolution limit of the SEM instrument used, which was estimated to be 10 nm. Also, we have performed a theoretical estimation of the vibration amplitude by modelling the capacitance between the NWs and the actuation electrode. Our estimations provide values of the order of 1 nm, which is consistent with previously reported estimations for similar devices electrostatically driven in similar conditions [2] , [3] . Although these qualitative considerations only set an upper limit for the amplitude of around 10 nm and a typical order of magnitude of around 1 nm, they show that the vibration amplitude a n is typically much smaller than the maximum deflection at rest d 0 . Electromechanical transduction signals in SiNW resonators In this section we compare the magnitude of the linear and quadratic components of the transduced signals. First, we show that the two-source/1 ω set-up is sensitive to signals arising from a linear transduction, whereas the two-source/2 ω detects the signals originated from the quadratic contribution. By comparing both responses under equal actuation conditions, the magnitude of the gain factor γ can be evaluated. The current through the resonator as a function of the change of resistance is: where V NW is the voltage applied to the SiNW and R NW is the total resistance. This approximation is valid when Δ R / R u ≪ 1, and here we estimate typically Δ R / R u ≈10 −3 . The above expression indicates that mixing occurs in general via multiplication of the terms V NW ( t ) and Δ R ( t ). Each of the down-mixing schemes uses a different signal for V NW ( t ) to mix with the different components of Δ R ( t ) given by equation (4), and then produce low-frequency components of the motional current that can be detected by a lock-in amplifier. The motional contribution to the current assuming piezoresistive transduction can thus be expressed by combining equations (4) and (6) as: For the two-source/1 ω and two-source/2 ω detection schemes, V NW ( t ) is a harmonic signal at frequencies ω+ω L and 2 ω+ω L , respectively: Therefore, mixing with the resonator vibration produces low-frequency signals at frequency ω L that for each case can be written as: The ratio of signal level between the two methods is equal to the enhancement factor defined in equation (4). If we assume a beam vibration in the fundamental mode ( n =1) (ref. 11 ) and a beam deflection profile shape at rest that can be approximated by that of the fundamental mode, then equations (10) and (11) can be rewritten as: so that the ratio between both signals is given by . The estimations provided above for the deflection at rest and vibration amplitude, with d 0 in the range of 5–50 nm and a 1 in the order of 1 nm, result in a ratio above 20. 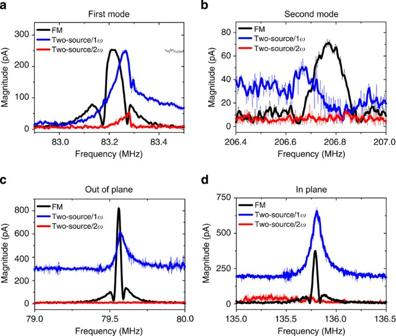Figure 3: Measurement of the frequency response of SiNW mechanical resonators obtained by the two-source/1ωand two-source/2ωdetection methods. (a,b) Bottom-up SiNW with a cross-sectional flat-to-flat distance of 52–60 nm and a length of 2.3 μm. (a) First mode, measurement conditions:VNW=36 mV,Vg,DC=7 V,Vg,AC=140 mV. (b) Second mode, measurement conditions:VNW=80 mV,Vg,DC=22 V,Vg,AC=140 mV. (c,d) Top-down SiNW with cross-sectional dimensions of 110 nm × 80 nm and a length of 3 μm. (c) In-plane vibration, measurement conditions:VNW,2source=80 mV,Vg,DC=10 V,Vg,AC=140 mV. (d) Out-of-plane vibration, measurement conditions:VNW,2source=80 mV,Vg,DC=15 V,Vg,AC=140 mV. Figure 3a,b shows the frequency response of a bottom-up SiNW with a cross-sectional flat-to-flat distance of 52–60 nm using the two-source/1 ω and two-source/2 ω detection schemes. We show the spectra for the first ( Fig. 3a ) and second ( Fig. 3b ) modes. The actuation conditions are equal for both methods, and therefore it can be assumed that the vibration amplitude is similar regardless of the detection method employed. We observe that the electrical signal amplitude is 3–14 times smaller for the two-source/2 ω , in agreement with the theoretical estimation provided above. Measurements of the dependence of the frequency response of the NW as a function of the constant (DC) gate voltage confirm that the electrical transduction generates a signal linearly proportional to the vibration amplitude in the case of the two-source/1 ω method and quadratic in the case of the two-source/2 ω (see Supplementary Fig. 6 ). Figure 3: Measurement of the frequency response of SiNW mechanical resonators obtained by the two-source/1 ω and two-source/2 ω detection methods. ( a , b ) Bottom-up SiNW with a cross-sectional flat-to-flat distance of 52–60 nm and a length of 2.3 μm. ( a ) First mode, measurement conditions: V NW =36 mV, V g,DC =7 V, V g,AC =140 mV. ( b ) Second mode, measurement conditions: V NW =80 mV, V g,DC =22 V, V g,AC =140 mV. ( c , d ) Top-down SiNW with cross-sectional dimensions of 110 nm × 80 nm and a length of 3 μm. ( c ) In-plane vibration, measurement conditions: V NW,2source =80 mV, V g,DC =10 V, V g,AC =140 mV. ( d ) Out-of-plane vibration, measurement conditions: V NW,2source =80 mV, V g,DC =15 V, V g,AC =140 mV. Full size image Figure 3c,d shows the measurement of the first mode of a top-down NW using the two-source/1 ω and two-source/2 ω detection schemes in the out-of-plane ( Fig. 3c ) and in-plane ( Fig. 3d ) directions. The SiNW has cross-sectional dimensions of 110 nm (width) × 80 nm (thickness), comparable to those of bottom-up NWs. As in the case of Fig. 3a,b , we employ the same actuation conditions for both detection methods, so the mechanical oscillation amplitude of the resonator is expected to be the same. It is noticeable that no resonance is detected using the two-source/2 ω method, indicating that for top-down devices the ratio between 1 ω and 2 ω signals is larger than 20, as estimated above. Similar results are obtained with smaller top-down NWs with a cross-section of 60 nm (thickness) × 72 nm (width), which are shown in Supplementary Fig. 7 . This indicates the absence (or very weak) quadratic transduction in top-down SiNWs under the current fabrication conditions. Measurements of the dependence of the frequency response of the vibration amplitude as a function of the gate voltage show that the electrical transduction generates a signal proportional to the amplitude when using the FM and two-source/1 ω methods (see Supplementary Fig. 8 ). In addition to piezoresistance, another possible alternative mechanism responsible for the linear transduction could be conductance modulation due to capacitive coupling induced by the side gate, similar to CNT and graphene resonators [1] , [28] , which has also been reported for top-down SiNWs [3] . However, we discard this mechanism for the devices under consideration here. Static transconductance measurements were performed in bottom-up SiNW nanomechanical resonators for gate voltages from −25 to 25 V (see Supplementary Fig. 9 ). They show a null or very weak conductivity modulation effect, as it is expected from the high doping level of the SiNWs and the large-gap distance between the gate and the SiNW. In consequence, the signal that originated from capacitive coupling would be much lower than the signal experimentally obtained by the FM and two-source/1 ω detection methods. The expected signal that should be measured by assuming conductance modulation by capacitive coupling would be of 4 pA, almost two orders of magnitude smaller than the one obtained experimentally ( Fig. 3a ). In the case of the top-down-fabricated devices, it is also found that the static and dynamic transconductance is very low, as no appreciable resistance change was observed during static transconductance measurements when varying the gate voltage from −25 to 25 V, and therefore a transduction mechanism based on capacitive coupling cannot explain the high level of the detected signals. We estimate a value for the transconductance of 20 nS V −1 from the purely electrical signal measured at a frequency far away from resonance using the two-source/1 ω method, which discards also the conductance modulation due to charge induced by the side gate as transduction mechanism (see Supplementary Fig. 10 ). The electrical signals obtained with the devices presented here are thus consistent with a purely piezoresistive transduction mechanism that produces linear and quadratic components in the dependence of the resistance variation with the vibration amplitude. From equations (12) and (13) and the estimations made for the deflection at rest and first-mode vibration amplitude ( a 1 ≈1 nm, d 0 =5–50 nm), we infer gauge factor values in the range from a few units to a few hundreds. This is the range expected from a conventional piezoresistive effect in SiNWs depending on the doping level [24] . Therefore, high-sensitivity piezoresistive transduction, enhanced by an asymmetric beam profile at rest, does not require extraordinarily large piezoresistive coefficients as those reported on high-resistivity bottom-up NWs, which reach up to 1,000 and above [21] . Nevertheless, larger gauge factors are still expected for bottom-up NWs as compared with their top-down counterparts according to the literature [23] , [24] . In fact, a larger gauge factor for bottom-up SiNWs explains why the quadratic component of the resistance variation with vibration is only detected for these devices ( Fig. 3 ). According to our model, while the deflection at rest represents a gain factor that allows to obtain a large linear transduction regardless of G , it does not modify the quadratic transduction, which depends only on G . In the experiments, bottom-up SiNW resonators provide measurable quadratic transduction signals at least for the first mode ( Fig. 3a ), whereas no quadratic detection is obtained for top-down SiNWs for any mode or vibration plane. This observation is consistent with the lower gauge factor for top-down SiNWs, which implies that the quadratic signal level is below the minimum detectable level in our set-up. However, the larger gauge factor of the bottom-up SiNWs does not necessarily imply larger linear signals than those of top-down devices because a larger deflection at rest of the later compensates for their lower piezoresistivity. Finally, we remark that our analysis assumes a linear dependence of the resistance variation with the strain. However, the initial strain caused by the asymmetric beam deflection at rest may lead to the onset of some nonlinearity in this dependence, but the fact that the vibration amplitude is very small makes it reasonable to consider a linear dependence for the strain variations caused by such vibrations. And remarkably, even in the case of a nonlinear variation of resistance with strain, an asymmetric beam profile at rest originates a signal that has a linear dependence with the vibration amplitude (see Supplementary Discussion ). In summary, we have described an enhanced piezoresistive transduction mechanism arising from an asymmetric beam shape at rest in doubly clamped SiNW resonators. Regardless of the detection scheme, this asymmetry introduces a linear component in the resistance variation that is proportional to the product of the vibration amplitude and to the magnitude of deflection at rest, while the quadratic component remains independent of this effect. When the deflection at rest is much larger than the vibration amplitude, this asymmetry produces a largely amplified linear response with respect to the quadratic one. This simultaneous linearization and amplification of piezoresistive transduction in Si beam resonators presents crucial implications for practical development of device applications. For instance, it enables detection of multiple modes at very high resonance frequencies that otherwise would not be easily detectable. Note that the detected high-order modes were electrostatically driven by side gates with a geometry not particularly optimized for the expected mode shapes. Multiple-mode detection has recently shown to be crucial for simultaneous measurements of mass and adsorption position of biomolecules for mass-sensing applications [4] and to quantum non-demolition measurements of the amplitude, making use of the inter-modal coupling [29] , [30] . In addition, a linear transduction mechanism allows to perform measurements using standard electrical methods, such as network analysers, as well as its incorporation in closed-loop oscillator topologies, both of which would be impaired by quadratic transduction. It should also be noted that an asymmetric beam shape in doubly clamped beams of nanometric dimensions is by no means an uncommon phenomena. In CNT resonators, it has been recently shown that such asymmetries are responsible for some particular features of their electromechanical response [31] . In the case of Si beams, top-down fabrication methods can be engineered to predetermine the amount of beam deflection at rest to target specific read-out signal levels. The transduction mechanism described here is indeed particularly relevant for top-down-fabricated Si resonators. The lack of an effective transduction mechanism was a limiting factor for exploiting the VLSI fabrication technologies available for such devices. The fact that the mechanism described here does not require exceptionally large piezoresistive factors or any other special material property different than those of doped bulk Si allows its immediate application for devices fabricated by VLSI techniques. Fabrication of bottom-up SiNWs The bottom-up fabrication method is based on the VLS growth mechanism catalysed by gold nanoparticles, which is described in more detail in ref. 32 and depicted in Fig. 4a . The process is performed on silicon-on-insulator (SOI) wafers. First, contacting pads, clamping structures and trenches are defined in the SOI layer using photolithography and dry etching. The wafers are cut into chips, each chip containing 392 structures where the nanomechanical resonator will be formed if the SiNW grows at the proper place. Catalyst particles are randomly deposited on the surface of the chip from a gold colloid solution. Then, the SiNWs are grown in the substrates using the VLS method in an atmospheric chemical vapour deposition. As a final step, the devices are doped by annealing the chips in close proximity to a fragment of a boron nitride wafer, so that the final resistivity of the SiNWs is very low in the range of 10 −4 Ω m. Two terminal characterization of released devices show a linear I / V curve and a typical resistance of 50 kΩ. Using this process, we have obtained resonators made of SiNWs with cross-sectional flat-to-flat distance in the range 50–100 nm and length of 1–3 μm. Some devices incorporate a silicon electrode close to the SiNW for electrostatic actuation. Typically, the gap distance between the gate and the SiNW is around 400 nm. Owing to the random placement of the catalyst material, the fabrication yield is relatively low: based on post-growth characterization, we have found it to be of roughly 5%, good enough to get a sufficient number of operative devices per chip. 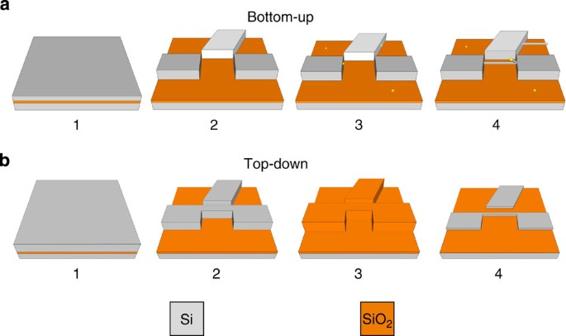Figure 4: Fabrication of nanomechanical resonators. (a) Bottom-up fabrication process. (1) SOI wafers are used as a substrate. (2) Clamping and pad structures are defined using photolithography and reactive ion etching. (3) Gold colloids are randomly deposited on the substrate. (4) SiNWs are grown using a chemical vapour deposition–VLS process. (b) Top-down fabrication process. (1) SOI substrate. (2) Pattern definition in the silicon device layer by photolithography and dry etching. (3) Oxidation to reduce the dimensions of the section of the resonator. (4) Oxide etching by hydrofluoric acid. Figure 4: Fabrication of nanomechanical resonators. ( a ) Bottom-up fabrication process. (1) SOI wafers are used as a substrate. (2) Clamping and pad structures are defined using photolithography and reactive ion etching. (3) Gold colloids are randomly deposited on the substrate. (4) SiNWs are grown using a chemical vapour deposition–VLS process. ( b ) Top-down fabrication process. (1) SOI substrate. (2) Pattern definition in the silicon device layer by photolithography and dry etching. (3) Oxidation to reduce the dimensions of the section of the resonator. (4) Oxide etching by hydrofluoric acid. Full size image Fabrication of top-down SiNWs An overview of the fabrication process is shown in Fig. 4b . An SOI wafer is used as a starting substrate. The patterns are defined using optical photolithography (i-line stepper), and then transferred to the silicon device layer using reactive ion etching. At this step, SiNWs with cross-sectional areas from 350 to 500 nm are obtained corresponding to the minimum feature size obtainable with the optical photolithography equipment. To reduce their cross-sections, an oxidation process is performed at 1,000 °C in an O 2 environment. Afterwards the oxide is removed by a dip in a solution with hydrofluoric acid followed by critical point drying. This cycle is repeated several times until the desired dimensions are obtained. Finally, the SiNWs are doped by performing an annealing in close proximity to a boron nitride wafer, as in the case of the bottom-up. Using this processing sequence, SINWs of dimensions comparable to their bottom-up counterparts are fabricated with high yield. By adjusting the oxidation steps, we have succeeded in fabricating SiNWs with a range of cross-sectional dimensions from 60 to 175 nm, and length of ~\n3 μm. Some devices incorporate a silicon electrode close to the SiNW for electrostatic actuation. Typically, the gap distance between the gate and the SiNW is around 900 nm. Electrical detection methods Electrical detection is performed by down-mixing radio-frequency methods, in which the high-frequency-transduced signal arising from the motion of the resonator is transferred to lower frequencies, and then detected using a lock-in amplifier. The measurements are performed in a vacuum chamber, at a pressure of 1 × 10 −6 mbar and at room temperature. Three electrical detection set-ups based on three different down-mixing methods have been employed in this work: the two-source/1 ω (ref. 1 ); the two-source/2 ω (ref. 2 ); and the FM demodulation [8] . Schemes of the experimental set-up for each detection method are shown in Fig. 5 , and a full description can be found in ref. 33 . 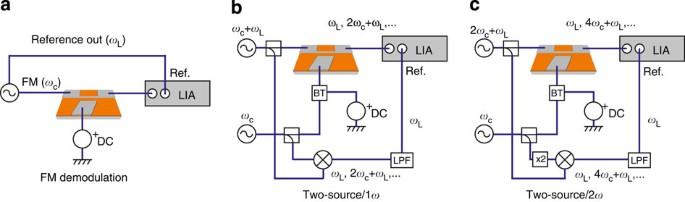Figure 5: Schematic of the electrical detection methods used in this work. (a) FM detection method. (b) Two-source/1ωdetection method. BT, Bias-Tee; LPF, low-pass filter; LIA, lock-in amplifier. (c) Two-source/2ωdetection method. Figure 5: Schematic of the electrical detection methods used in this work. ( a ) FM detection method. ( b ) Two-source/1 ω detection method. BT, Bias-Tee; LPF, low-pass filter; LIA, lock-in amplifier. ( c ) Two-source/2 ω detection method. Full size image How to cite this article : Sansa, M. et al. High-sensitivity linear piezoresistive transduction for nanomechanical beam resonators. Nat. Commun. 5:4313 doi: 10.1038/ncomms5313 (2014).